The use of referential gestures in ravens (Corvus corax) in the wild Around the age of one year, human children start to use gestures to coordinate attention towards a social partner and an object of mutual interest. These referential gestures have been suggested as the foundation to engage in language, and have so far only been observed in great apes. Virtually nothing is known about comparable skills in non-primate species. Here we record thirty-eight social interactions between seven raven ( Corvus corax ) dyads in the Northern Alps, Austria during three consecutive field seasons. All observed behaviours included the showing and/or offering of non-edible items (for example, moss, twigs) to recipients, leading to frequent orientation of receivers to the object and the signallers and subsequent affiliative interactions. We report evidence that the use of declarative gestures is not restricted to the primate lineage and that these gestures may function as 'testing-signals' to evaluate the interest of a potential partner or to strengthen an already existing bond. From early childhood on, human infants frequently use distinct gestures such as showing, offering, giving (for example, food, objects), and pointing [1] to coordinate attention towards a social partner and an object of mutual interest [2] . These triadic interactions qualify as referential because they are used to attract the attention of others to some outside entity, are mechanically ineffective and include joint-attention behaviours (for example, eye-contact with an adult before, during or after the performance of a gesture). They are used either to make requests (imperatives, for example, 'take this') or to show a third entity to recipients, without requiring the person to do anything else but to attend to the object (declaratives, for example, 'look at this') [3] . These gestures thus mark a pivotal change in the infant's communicative competence and have been viewed as the foundation to engage in symbolically mediated conversations [1] , [4] . In stark contrast, observations of comparable gestures in our closest living relatives, the great apes, are relatively rare and mainly concern captive and/or human-raised individuals [5] , [6] , [7] , [8] , [9] , [10] . The most compelling evidence of referential gestures in natural environments so far stems from chimpanzees at the Ngogo community, Uganda, who use so-called directed scratches, to indicate distinct spots on their bodies to be groomed [11] . These attention-getters represent, due to their two-tiered intentional structure (combining social intention to get something done and the 'referential' intention to draw the attention of the recipient to some third entity), an extremely rare form of communication evolutionarily and have been suggested as confined to primates only [12] . However, are such sophisticated gestures truly unique to the primate lineage? In the present study, we aimed to address this question by investigating the use and underlying cognitive complexity of distinct nonvocal signals in ravens ( Corvus corax ) in their natural environment. Ravens are songbirds, which show a relatively high degree of song learning, including the ability to mimic the songs of other birds and human speech, along with environmental sounds [13] , [14] . Although Gwinner [14] in the middle of the last century, already emphasized their gestural plasticity and flexibility, research into this communicative domain is virtually nonexistent. Ravens belong to the corvid family, which is renowned for exceeding the majority of other avian species with the exception of some parrots, [15] , [16] and rivalling even primates in many physical and social cognitive domains (for example, see refs 17 , 18 and 19 ). Unlike nonhuman primates, but similarly to humans, corvids rely heavily on cooperation between pair-partners [14] , [20] . Ravens in particular can be characterized by ontogenetically shaped intra-pair communication [14] , [20] , [21] , relatively long-time periods to form pairs [14] , [20] , [22] , and variation in relationship quality within non-breeder groups [23] . Moreover, ravens often use non-food items in social interactions [20] , [24] . The motives to form and maintain affiliate relationships may, thus, have been crucial in boosting not only their cognitive but also, especially, their vocal and nonvocal communicative abilities. Notably, first stages of social bonding may involve behaviours to direct other's attention triadically and referentially [25] . Our results provide evidence that the use of referential gestures is not restricted to the primate lineage. Ravens also use distinct object-oriented behaviours to mainly direct conspecific's attention to a third entity triadically and referentially. As the majority of gestures were used in mixed-sex dyads, these gestures seem to function as 'testing-signals' to evaluate the interest of a given partner or to strengthen an already existing bond. Our results thus support the hypothesis that evolutionary new inferential processes ensue when communication becomes governed by more cooperative motives [26] , and that examples of convergent evolution in distant-related species provide crucial clues to unravel the mystery of language origins. 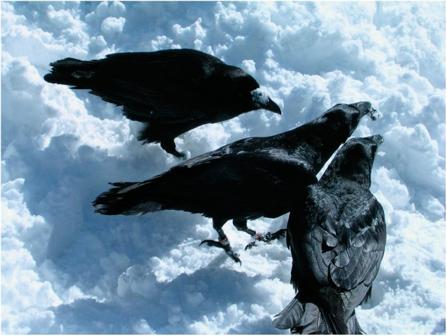Figure 1: Showing. Raven showing an object to conspecifics. Gesture use We recorded 38 social interactions of 7 raven dyads in their natural habitat ( Table 1 ). Eight of twelve possible interactants were tagged and could clearly be identified. Four individuals were untagged and, based on their morphology and behaviour, could only be clustered in relation to their age, but not sex class. The four dyads, which consisted of tagged individuals consisted all of mixed-sex pairs. All dyads engaged in two distinct behaviours, showing and offering. Twenty-five instances consisted of showing, defined as 'picking up a non-food item (for example, moss, small stones, or twigs), holding it up in the beak, head straight or tilted upwards, and staying in this position ( Fig. 1 )'. Ten instances consisted of offering, defined as 'picking up a non-food item (for example, moss, small stones, or twigs), holding it up in the beak and moving the head up- and/or downwards repeatedly' ( Table 1 ). Table 1 Individuals, age, recipients, behavioural parameters. Full size table Figure 1: Showing. Raven showing an object to conspecifics. Full size image In the majority of the observed cases, these behaviours were directed to a recipient (100%), were mechanically ineffective (that is, they were not designed to act as direct physical agents, contrary to behaviours such as sticking an object in the beak of a given recipient) (95%), and received a voluntary response (100%). Concerning the underlying cognitive complexity [27] , the analyses showed that the behaviours were followed by response waiting (100%), and were, significantly, more often directed to an attending recipient than to a non-attending recipient (Wilcoxon test: Z =−2.371, n =7, exact P -value=0.018; Fig. 2 ). 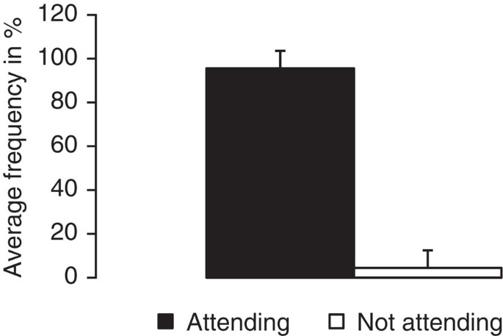Figure 2: Adjustment to audience effects. Average use (in %) of showing and offering (collapsed) to an attending and non-attending recipient. Error bars indicate the s.d. Figure 2: Adjustment to audience effects. Average use (in %) of showing and offering (collapsed) to an attending and non-attending recipient. Error bars indicate the s.d. Full size image Orientation of recipients and subsequent behaviour of dyad In addition, after the performance of a signal recipients oriented themselves significantly more often towards the signaller and the object than away from them (Wilcoxon test: Z =−2.375, n =7, exact P -value=0.018; Fig. 3 ). In the majority of cases, recipients engaged subsequently in affiliative interactions with the signaller (approaching, billing, pretend-feeding, manipulating of the object together: 77%), and only rarely in agonistic/defensive (4%) or more neutral interactions (other behaviour: vocalizing, ignoring: 11%; change of attentional state from non-looking to looking: 8%). These differences were significant for affiliative versus agonistic/defensive behaviour (Friedman X 3 2 =15.879, P =0.001; Wilcoxon test: Z =−2.375, n =7, post-hoc corrected P -value (Holm)=0.036; Fig. 4 ). 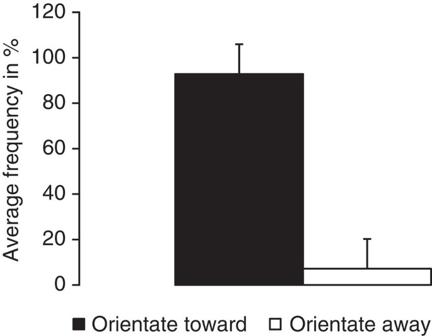Figure 3: Orientation of the recipient after performance of showing and offering. Average orientation of the recipient (in %) towards and away from the signaller after the performance of showing and offering (collapsed). Error bars indicate the s.d. Figure 3: Orientation of the recipient after performance of showing and offering. Average orientation of the recipient (in %) towards and away from the signaller after the performance of showing and offering (collapsed). Error bars indicate the s.d. 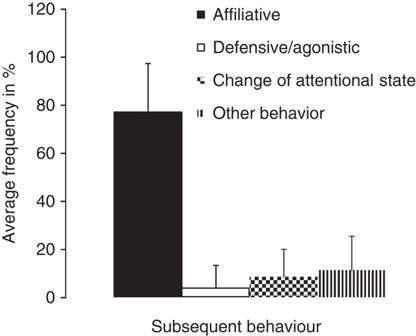Figure 4: Subsequent behaviour in dyads after performance of showing and offering. Average frequency (in %) of either affiliative (approaching, billing, manipulating the object together), defensive/agonistic behaviour (defensive posture, leave, flee, attack), attentional state changes (from non-looking to looking) or other behaviour (vocalizing, ignoring) between members of the dyad after the performance of showing and offering (collapsed). Error bars indicate the s.d. Full size image Figure 4: Subsequent behaviour in dyads after performance of showing and offering. Average frequency (in %) of either affiliative (approaching, billing, manipulating the object together), defensive/agonistic behaviour (defensive posture, leave, flee, attack), attentional state changes (from non-looking to looking) or other behaviour (vocalizing, ignoring) between members of the dyad after the performance of showing and offering (collapsed). Error bars indicate the s.d. Full size image The present study aimed to investigate whether members of the corvid family, ravens, use nonvocal signals as sophisticated, referential means. Our results showed that ravens used distinct object-oriented behaviours, showing and offering, to already attending recipients of the opposite sex. In response to these behaviours, recipients oriented themselves most often directly towards the object and the signaller and engaged, subsequently, more often in affiliative behaviour with the signaller (including behaviours such as billing and manipulating of the object) than in agonistic or defensive behaviour. Three hypotheses may account for these observations. First, showing and offering may not serve a communicative function, but may be due to the predisposition of especially young individuals to explore and manipulate almost every kind of object they encounter [28] . It has been suggested that the manipulation and exploration of objects may serve to familiarize young ravens with potential food items that may be unique to their ecological circumstances [28] . Furthermore, ravens like other food-storing corvids devote much of their time to cache food in temporary storages [29] . They are also known for caching small non-food items [30] , suggesting that they 'enjoy' hiding items and, in the absence of food, become directed towards objects. This hypothesis suggests that showing and offering takes place irrespectively of the presence and attentional state of a given recipient. These two predictions do not accord with our observations ( Figs 1 and 2 ). Second, showing and offering may not represent communicative signals but are simply due to the intrinsic motivation [31] to share food [20] . Contrary to nonhuman primates, active giving or allofeeding is very common in birds, especially with regard to parent–offspring [32] and courtship feeding [33] , [34] . This motivation may be so strong that the birds perform the behaviour even if no food is available. If this hypothesis was true, then we would expect that ravens only offer, but not show objects, to recipients and that all interactions end in attempts to allofeed the recipient. However, we only observed once that a raven that had offered a piece of moss to a recipient, tried to subsequently put it in the beak of the recipient. In addition, we did not observe any other characteristic behaviours such as twitching of the wings and feeding vocalizations, which have been described to accompany allofeeding [14] , [20] . Third, showing and offering may be used communicatively to direct others' attention intentionally to external things triadically and referentially. Consistent with this hypothesis is that both behaviours were always directed to a recipient, were mechanically ineffective, received a voluntary response, and showed goal-directedness and sensitivity to the attentional state of recipients. These signals thus qualify, following the criteria of Bates and colleagues [3] and Pika [27] as intentionally produced communicative gestures and are understood by receivers. Our observations thus strengthen the findings of Gwinner [14] , who suggested a high degree of flexibility in ravens' nonvocal signalling. Interestingly, the only other study suggesting referential gestural abilities in birds, concerns another highly social and cooperative songbird belonging to the family of the Artamidae [35] . Kaplan [36] reported that Australian magpies ( Gymnorhina tibicen ) show a distinct body posture when encountering a sheltered or partly hidden aerial raptor, the wedge-tailed eagle ( Aquila audax ): they lean forward in an angle of nearly 45° below a normal resting position, while the body is forming a straight line with the beak facing the eagle. Because additionally arriving Australian magpies engaged in gaze following, when landing and quite often also adopted the same posture, Kaplan argued that this behaviour qualifies as a proto-declarative act of 'pointing' to change the state of knowledge of another conspecific (for a critical evaluation of the use of the term proto-declarative for non-linguistic species, refs 5 , 37 ). However, as the majority of arriving magpies adopt the same posture, the signal might, in fact, be aimed at the predator itself rather than serving to inform conspecifics [38] , [39] . Further research is needed to investigate whether Australian magpies and other highly social and cooperative bird species use nonvocal signals as intentionally produced strategies to inform conspecifics about third entities and/or events. In sum, our results provide the first evidence that ravens, similarly to pre-linguistic human children and great apes, use nonvocal signals to direct the attention of conspecifics to outside entities triadically and referentially (for ravens' functional referential vocal abilities, ref. 40 ). However, contrary to chimpanzees, whose referential gestures to conspecifics are requests for distinct activities (for example, 'groom me here') and are directed to partners of both sexes [11] , [41] , ravens' referential gestures seem mainly be performed towards members of the opposite sex and may thus function as 'test signals'. As ravens rely heavily on cooperation between pair-partners to raise their young and bond for life [20] , they invest in relatively long time periods to find and choose the right partner. Gestures such as showing and offering might thus have developed in this object-oriented species, to explore whether a given partner would be interested in attending to oneself and a given object of interest; and/or to test and strengthen an already existing relationship. The function of these gestures may, thus, be very similar to declarative gestures (used to share attention or to comment on things) of pre-linguistic human children such as pointing and showing, which are most frequently used between individuals with already existing strong bonds (for example, mother–infant) or in situations of uncertainty, in which bonds just have to be formed (for example, meeting of strangers) [25] . The use of triadic referential signals in wild ravens thus adds to the growing evidence that corvids are in many cognitive domains comparable to nonhuman primates and may even exceed them in some [42] , [43] . Furthermore, because ravens, like humans, rely heavily on cooperation between pair-partners [20] , our results strengthen the hypothesis that evolutionary new inferential processes ensue when communication becomes governed by more cooperative motives [26] . To reconstruct hominid evolution and the changes that paved the way for language to evolve, we thus have to view the likely adaptations of early hominins generally, rather than with specific reference to living chimpanzees only [44] . Detailed insight in communicative abilities of our closest phylogenetic relatives, the nonhuman primates, can, by both homology and analogy, help in reconstructing the behaviour of the last common ancestor of Pan and Homo and, perhaps, some aspect of early hominin behaviour. Examples of convergent evolution in distant-related species, however, will provide crucial clues to the types of problems that particular morphological or behavioural mechanisms were 'designed' to solve [45] . Data collection We observed individually marked members ( Table 1 ) of a wild raven community in Northern Alps, Austria, which are habituated to human observers at foraging and socializing sites within areas of the Cumberland Wildpark, Grünau. Observations were carried out on 68 days, outside the breeding season during three consecutive field periods (September 2008, June–August 2009 and June 2010). Communicative behaviour was recorded on an opportunistic basis (sampling rule: behaviour sampling; recording rule: continuous recording, Martin & Bateson, 1994), using a HD-camera (Sony HDR-CX11E HD Camcorder) and a Personal digital assistant. Gestural definition Following the primate literature [27] , gestures were defined as movements of the limbs or head and body that are directed towards a recipient, are goal-directed, mechanically ineffective (that is, they are not designed to act as direct physical agents) and receive a voluntary response. The following behavioural criteria were used to infer goal-directedness: gazing at the recipient, and response waiting (the signaller waits for a response after the signal has been produced). Data coding, reliability and statistical analyses The digital videotapes were transferred to a computer and cut into salient segments. The data collected with the Personal digital assistant were also transferred to a computer. All data were coded using the program Adobe Premiere 7 and/or Excel. Ten percent of the data set was coded for accuracy by a second observer, resulting in a Cohen's Kappa of 0.82, an excellent level of agreement [46] . Non-parametrical tests were applied to carry out statistical analyses, followed by post-hoc-tests for several pairwise-comparisons (Holms). How to cite this article: Pika, S. & Bugnyar, T. The use of referential gestures in ravens ( Corvus corax ) in the wild. Nat. Commun. 2:560 doi: 10.1038/ncomms1567 (2011).